Epidermal phospholipase Cδ1 regulates granulocyte counts and systemic interleukin-17 levels in mice Phospholipase C is a key enzyme in phosphoinositide turnover. Although its functions have been extensively studied at the cellular level, many questions remain concerning its functions at the organ and individual animal levels. Here we demonstrate that mice lacking phospholipase Cδ1 develop granulocytosis associated with elevated serum levels of the granulopoietic cytokine interleukin-17. Re-introduction of phospholipase Cδ1 into keratinocytes of phospholipase Cδ1 -deficient mice reverses this phenotype, whereas conditional ablation of phospholipase Cδ1 in keratinocytes recreates it. Interleukin-17 and its key upstream regulator interleukin-23 are also upregulated in epidermis. Loss of phospholipase Cδ1 from keratinocytes causes features of interleukin-17-associated inflammatory skin diseases. Phospholipase Cδ1 protein is downregulated in the epidermis of human psoriatic skin and in a mouse model of psoriasis. These results demonstrate that phosphoinositide turnover in keratinocytes regulates not only local inflammatory responses but also serum cytokine levels and systemic leukocyte counts, and affects distant haematopoietic organs. Phospholipase C (PLC) is a key enzyme in phosphoinositide turnover, an important signal transduction process in cells. PLC hydrolyses phosphatidylinositol 4,5-bisphosphate (PIP 2 ) to generate the second messengers inositol 1,4,5-trisphosphate (IP 3 ) and diacylglycerol (DAG), leading to elevated intracellular calcium ion concentrations and activation of protein kinase C (PKC) [1] , [2] . Although the functions of PLC have been extensively studied at the single-cell level [3] , its physiological role in interactions among different cell types in vivo remains largely unknown. Humoural factors communicate between different, distantly located cell types, and induce various physiological and cellular events such as inflammation, cell growth and apoptosis. Cytokines are one type of such humoural factors. Interleukin (IL)-17, also called IL-17A, is a pleiotropic cytokine that has emerged as a central player in the mammalian immune system, with important roles in the pathology of many disease processes, including allergic responses [4] and autoimmune diseases [5] , [6] , [7] , [8] , [9] , [10] . IL-17 is mainly produced by T lymphocytes under the regulation of IL-23 (refs 11 , 12 ), and in turn, regulates granulopoiesis through induction of granulocyte colony-stimulating factor (G-CSF) [13] , [14] , [15] . Granulocytes are key players in the pathogenesis of several inflammatory diseases. Increased baseline circulating granulocyte number is a risk factor for all-cause mortality and the progression of chronic diseases such as atherosclerosis and chronic renal failure [16] , [17] , [18] . We previously reported that one of the PLC isozymes, PLCδ1, was abundantly expressed in the epidermis [19] and that systemic loss of PLCδ1 resulted in epidermal hyperplasia associated with the infiltration of immune cells [20] . The epidermis is mainly composed of keratinocytes and is characterized by a polarized pattern of epithelial growth and differentiation, with a single basal layer of proliferating keratinocytes and multiple, overlying differentiated layers. Epidermal keratinocytes not only act as a barrier to the external environment, but also exert important functions in skin immune responses by secreting a variety of cytokines that initiate local inflammatory responses [21] . Indeed, keratinocytes have pivotal roles in the pathogenesis of human inflammatory skin diseases, including psoriasis and atopic dermatitis [22] . However, little is known about the ability of keratinocytes to regulate systemic inflammatory responses. Here we demonstrate that loss of epidermal PLCδ1 results not only in skin inflammation associated with aberrant activation of IL-23/IL-17 axis, but also in systemic inflammation, characterized by increase in serum cytokine levels and systemic granulocytosis. Loss of systemic PLCδ1 causes granulocytosis Loss of PLCβ3 in haematopoietic cells alters blood cell counts and populations in a haematopoietic cell intrinsic manner [23] . As PLCβ3 binds to PLCδ1 (ref. 24 ) in a manner similar to the binding of PLCβ2, we investigated if the systemic loss of PLCδ1 also affected blood cell counts and populations. Mice lacking the PLCδ1 gene ( PLCδ1 −/− mice) exhibited a greater than twofold increase in peripheral blood leukocytes compared with wild-type mice (mean±s.e.m. cell numbers, 9.2±0.85×10 6 in wild-type versus 19±1.4×10 6 in PLCδ1 −/− mice, n =6 for wild-type and n =9 for PLCδ1 −/− mice). We also examined the population of CD11b + Gr-1 + granulocytes. At first, we confirmed that PLCδ1 +/− mice did not exhibit increase in granulocytes ( Supplementary Fig. S1 ), and PLCδ1 +/− mice were, therefore, used as a control in subsequent experiments. Granulocytes were markedly increased in the peripheral blood leukocyte in PLCδ1 −/− mice, as well as in the spleen and bone marrow ( Fig. 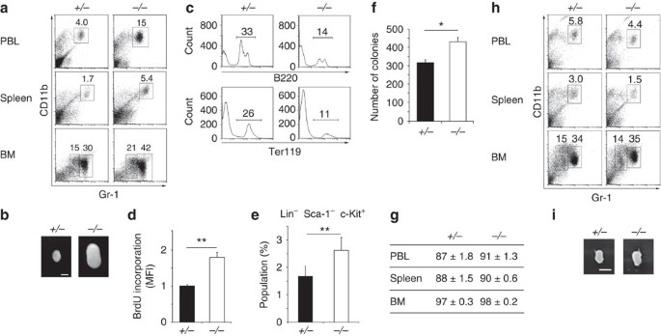Figure 1:PLCδ1−/−mice show granulocytosis in non-haematopoietic cell intrinsic manner. (a) Representative FACS profiles of CD11b+Gr-1+granulocytes in peripheral blood leukocytes (PBL), spleen, and bone marrow (BM) (n=14). Granulocytes in bone marrow were categorized into immature (CD11b+Gr-1low) and mature (CD11b+Gr-1high) subsets. (b) Macroscopic appearance of ILNs. Scale bar, 2 mm. (c) Representative FACS profiles of B220+and Ter119+cells in the BM (n=7–12). (d) BrdU incorporation in immature granulocytes (CD11b+Gr-1low) in the BM. Data are expressed as the relative mean fluorescence intensity (MFI)±s.e.m. (MFI ofPLCδ1+/−mice=1) (n=5). (e) Populations of myeloid progenitor-rich Lin−Sca-1−c-Kit+cells in the BM. Mean±s.e.m. (n=8). (f)In vitrocolony-forming assay. The numbers of colony-forming cells per 6×104cells at 12 days after plating are displayed. Mean±s.e.m. (n=4). (g) Haematopoietic chimerism analysis. Chimerism of the PBL, spleen, and BM were determined in transplanted mice by FACS analysis of CD45.1−cells. Mean percentage±s.e.m. Six recipients in each group. Three donor mice per genotype were used. (h) Representative FACS profiles of CD45.1−CD11b+Gr-1+granulocytes in the PBL, spleen, and BM of CD45.1+congenic recipients reconstituted withPLCδ1+/−orPLCδ1−/−BM at 4 weeks post-transplantation. (n=6). Plots shown are gated on CD45.1−cells. (i) Macroscopic appearance of the ILNs. Scale bar, 2 mm. Mice used in all experiments were 8–12 weeks old. Statistical significance was assessed using a Student′st-test. *P<0.05; **P<0.01. 1a ; Table 1 ). PLCδ1 −/− mice also showed lymphadenopathy of the inguinal lymph nodes (ILNs) and mild splenomegaly ( Fig. 1b ; Supplementary Table S1 ). We confirmed that expression of other PLC isoforms was not affected by loss of PLCδ1 ( Supplementary Fig. S2 ). Antibiotic treatment of PLCδ1 −/− mice had no effect on the development of granulocytosis and lymphadenopathy ( Supplementary Fig. S3a–d ), and PLCδ1 −/− granulocytes seemed to be morphologically and functionally normal ( Supplementary Fig. S4a–c ), suggesting that the observed granulocytosis was not a secondary effect of bacterial infection or impaired granulocyte function. Enhanced granulopoiesis in the bone marrow is often accompanied by a reduction of B lymphocytes and erythrocytes [25] , [26] , [27] , and reduced numbers of B220 + B lymphocytes and Ter119 + erythrocytes were indeed observed in the bone marrow of PLCδ1 −/− mice ( Fig. 1c ; Table 1 ). Granulocytes in mouse bone marrow can be categorized into immature and mature subsets [28] , both of which were elevated in PLCδ1 −/− bone marrow ( Fig. 1a ), suggesting that the increase in the granulocyte population arose from an immature progenitor population. A 5-bromo-2′-deoxy-uridine (BrdU) incorporation assay revealed that the proliferative activity of immature granulocytes was higher in PLCδ1 −/− than in PLCδ1 +/− bone marrow ( Fig. 1d ), suggesting that the increase in granulocyte number resulted from enhanced proliferation of immature granulocytes. An increased population of myeloid progenitor cells could also increase the granulocyte number in PLCδ1 −/− mice. Indeed, the population of myeloid progenitor cells was greater in the bone marrow of PLCδ1 −/− than of PLCδ1 +/− mice ( Fig. 1e ), as was the number of myeloid colony-forming units ( Fig. 1f ), indicating that the loss of PLCδ1 resulted in an increased population of myeloid progenitor cells in the bone marrow, possibly leading to granulocytosis. Figure 1: PLCδ1 −/− mice show granulocytosis in non-haematopoietic cell intrinsic manner. ( a ) Representative FACS profiles of CD11b + Gr-1 + granulocytes in peripheral blood leukocytes (PBL), spleen, and bone marrow (BM) ( n =14). Granulocytes in bone marrow were categorized into immature (CD11b + Gr-1 low ) and mature (CD11b + Gr-1 high ) subsets. ( b ) Macroscopic appearance of ILNs. Scale bar, 2 mm. ( c ) Representative FACS profiles of B220 + and Ter119 + cells in the BM ( n =7–12). ( d ) BrdU incorporation in immature granulocytes (CD11b + Gr-1 low ) in the BM. Data are expressed as the relative mean fluorescence intensity (MFI)±s.e.m. (MFI of PLCδ1 +/− mice=1) ( n =5). ( e ) Populations of myeloid progenitor-rich Lin − Sca-1 − c-Kit + cells in the BM. Mean±s.e.m. ( n =8). ( f ) In vitro colony-forming assay. The numbers of colony-forming cells per 6×10 4 cells at 12 days after plating are displayed. Mean±s.e.m. ( n =4). ( g ) Haematopoietic chimerism analysis. Chimerism of the PBL, spleen, and BM were determined in transplanted mice by FACS analysis of CD45.1 − cells. Mean percentage±s.e.m. Six recipients in each group. Three donor mice per genotype were used. ( h ) Representative FACS profiles of CD45.1 − CD11b + Gr-1 + granulocytes in the PBL, spleen, and BM of CD45.1 + congenic recipients reconstituted with PLCδ1 +/− or PLCδ1 −/− BM at 4 weeks post-transplantation. ( n =6). Plots shown are gated on CD45.1 − cells. ( i ) Macroscopic appearance of the ILNs. Scale bar, 2 mm. Mice used in all experiments were 8–12 weeks old. Statistical significance was assessed using a Student′s t -test. * P <0.05; ** P <0.01. Full size image Table 1 Absolute numbers of granulocytes, erythrocytes, and B and T lymphocytes in peripheral blood, spleen, bone marrow, and inguinal lymph nodes. Full size table As granulocytosis in PLCδ1 −/− mice was likely caused by the lack of PLCδ1 in the haematopoietic compartment, we generated mice lacking PLCδ1 in the haematopoietic compartment by bone marrow transfer. Surprisingly, mice transplanted with PLCδ1 −/− bone marrow did not develop granulocytosis or lymphadenopathy ( Fig. 1g–i ), indicating that the loss of PLCδ1 in the haematopoietic system was not responsible for these phenotypes, and that the mechanism of granulocytosis in PLCδ1 −/− mice differed from that in mice lacking PLCβ3 (ref. 23 ). PLCδ1 −/− mice display local and systemic IL-17 upregulation The granulocyte population was increased and the B220 + B lymphocyte and Ter119 + erythrocyte populations were decreased in the bone marrow of PLCδ1 −/− mice ( Fig. 1a,c ; Table 1 ). However, the balance among colony-forming unit (CFU)- granulocyte/erythroid/macrophage/megakaryocyte, -granulocyte/macrophage, -macrophage, -granulocyte, and burst-forming unit-erythroid (BFU-E) was not dramatically disrupted in PLCδ1 −/− bone marrow cells cultured in vitro ( Supplementary Fig. S5 ). We therefore speculated that granulocytosis in PLCδ1 −/− mice was induced by humoural factors secreted from peripheral tissues. IL-17 is a critical cytokine for granulopoiesis [13] , [14] , [15] , and we, therefore, assessed serum IL-17 concentrations. IL-17 levels in the serum of control mice were below the detection limit, but those in PLCδ1 −/− mice were detectable ( Fig. 2a ), indicating that circulating levels of the granulopoietic cytokine IL-17 were increased in PLCδ1 −/− mice. The concentrations of other granulopoietic factors were not increased in PLCδ1 −/− mice ( Supplementary Fig. S6 ), strongly suggesting that IL-17 elevation is responsible for granulocytosis in these mice. 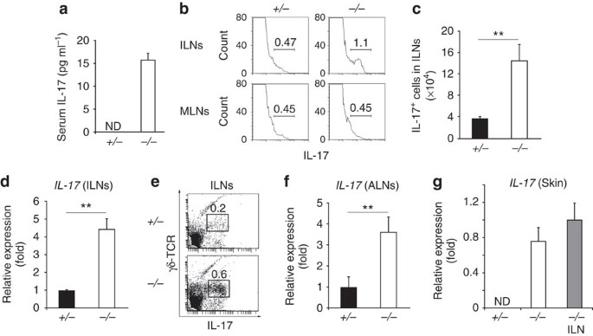Figure 2: Local and systemic IL-17 upregulation inPLCδ1−/−mice. (a) IL-17 concentration in the serum measured by ELISA. Mean±s.e.m. (n=6). (b) Representative FACS profiles of intracellular IL-17 in ILNs and MLNs. Cells were stimulated and intracellular IL-17 was detected (n=6 for ILNs andn=3 for MLNs). Three independent experiments were performed. (c) Absolute numbers of IL-17+cells in ILNs. Mean±s.e.m. (n=6). The combined results from three independent experiments are displayed. (d)IL-17mRNA expression in the ILNs determined by real-time RT–PCR. All values are normalized toglyceraldehyde 3-phosphate dehydrogenase(GAPDH). Results are displayed as arbitrary units (expression inPLCδ1+/−mice=1). Mean±s.e.m. (n=3). (e) Representative FACS profiles of γδ-TCR and intracellular IL-17 in ILNs (n=3). Cells were stimulated and intracellular IL-17 was detected. Three independent experiments were performed. (f)IL-17mRNA expression in the axillary lymph nodes (ALNs) determined by real-time RT–PCR. All values are normalized toGAPDH. Results are displayed as arbitrary units (expression inPLCδ1+/−mice=1). Mean±s.e.m. (n=5). (g)IL-17mRNA expression in skin determined by real-time RT–PCR.PLCδ1−/−ILN was used as the positive control forIL-17expression. All values are normalized toGAPDH. Results are displayed as arbitrary units (expression inPLCδ1−/−ILN=1). Mean±s.e.m. (n=5). Mice used in all experiments were 8–12 weeks old. Statistical significance was assessed using a Student′st-test. **P<0.01. ND; not detected. Figure 2: Local and systemic IL-17 upregulation in PLCδ1 −/− mice. ( a ) IL-17 concentration in the serum measured by ELISA. Mean±s.e.m. ( n =6). ( b ) Representative FACS profiles of intracellular IL-17 in ILNs and MLNs. Cells were stimulated and intracellular IL-17 was detected ( n =6 for ILNs and n =3 for MLNs). Three independent experiments were performed. ( c ) Absolute numbers of IL-17 + cells in ILNs. Mean±s.e.m. ( n =6). The combined results from three independent experiments are displayed. ( d ) IL-17 mRNA expression in the ILNs determined by real-time RT–PCR. All values are normalized to glyceraldehyde 3-phosphate dehydrogenase ( GAPDH ). Results are displayed as arbitrary units (expression in PLCδ1 +/− mice=1). Mean±s.e.m. ( n =3). ( e ) Representative FACS profiles of γδ-TCR and intracellular IL-17 in ILNs ( n =3). Cells were stimulated and intracellular IL-17 was detected. Three independent experiments were performed. ( f ) IL-17 mRNA expression in the axillary lymph nodes (ALNs) determined by real-time RT–PCR. All values are normalized to GAPDH . Results are displayed as arbitrary units (expression in PLCδ1 +/− mice=1). Mean±s.e.m. ( n =5). ( g ) IL-17 mRNA expression in skin determined by real-time RT–PCR. PLCδ1 −/− ILN was used as the positive control for IL-17 expression. All values are normalized to GAPDH . Results are displayed as arbitrary units (expression in PLCδ1 −/− ILN=1). Mean±s.e.m. ( n =5). Mice used in all experiments were 8–12 weeks old. Statistical significance was assessed using a Student′s t -test. ** P <0.01. ND; not detected. Full size image We investigated IL-17 production by lymphocytes in lymph nodes including ILNs and mesenteric lymph nodes (MLNs) by intracellular cytokine staining. The population of IL-17-producing cells was increased in ILNs, but not in MLNs, in PLCδ1 −/− mice ( Fig. 2b ). The number of IL-17-producing cells in the ILNs of PLCδ1 −/− mice exhibited a 3.9-fold increase compared with that in PLCδ1 +/− mice ( Fig. 2c ). IL-17 messenger RNA expression in ILNs, analysed using real-time RT–PCR was increased in PLCδ1 −/− mice ( Fig. 2d ). We then investigated the specific cellular source of IL-17 in ILNs of PLCδ1 −/− mice. Fluorescence-activated cell sorting (FACS) analysis revealed that the main producers of IL-17 were the γδ-T-cell receptor (TCR)-positive T cells ( Fig. 2e ). ILNs are skin-draining, whereas MLNs are not, suggesting that IL-17 was specifically upregulated in skin-draining lymph nodes. Indeed, another type of skin-draining lymph nodes, the axillary lymph nodes, also expressed high levels of IL-17 mRNA ( Fig. 2f ). These results suggest that the skin system has a pivotal role in IL-17 upregulation. Importantly, IL-17 expression was detected in PLCδ1 −/− skin, but not in normal skin ( Fig. 2g ). In contrast to IL-17, the expression of interferon γ and IL-4 was not increased in skin of PLCδ1 −/− mice ( Supplementary Fig. S7a ). Thus, PLCδ1 −/− mice showed IL-17 upregulation in skin and skin-draining lymph nodes. Epidermal PLCδ1 is sufficient for normal IL-17 levels Among skin cells, keratinocytes express the highest levels of PLCδ1 (ref. 19 ). In addition, IL-17 was upregulated in skin and skin-draining lymph nodes. We, therefore, hypothesized that the PLCδ1 in keratinocytes primarily regulates IL-17 levels. To test this hypothesis, we investigated whether reintroduction of PLCδ1 into keratinocytes of PLCδ1 −/− mice could restore normal IL-17 levels. We previously reported that expression of PLCδ1 in keratinocytes was mainly regulated by the transcription factor Foxn1 (ref. 29 ) and we, therefore, used a Foxn1 promoter-driven PLCδ1 gene ( Foxn1::PLCδ1 ) ( Fig. 3a ) to restore PLCδ1 expression in PLCδ1 −/− keratinocytes in a manner resembling that of endogenous PLCδ1 . Mice carrying Foxn1::PLCδ1 ( Fig. 3b ) appeared normal and did not exhibit any overt changes. Intercrossing PLCδ1 −/− mice and mice carrying Foxn1::PLCδ1 produced PLCδ1 −/− mice carrying Foxn1::PLCδ1 ( Tg/KO mice). PLCδ1 expression was restored in the skin of Tg/KO mice, but not in other organs such as the lungs, brain, ILNs, spleen and bone marrow ( Fig. 3c ). PLCδ1 protein was weakly expressed in Tg/KO thymuses, but these thymuses did not show obvious phenotypes, such as a disturbed balance of T-cell subtypes. Although the level of expression of PLCδ1 protein was somewhat lower in Tg/KO than in wild-type and heterozygous skin ( Supplementary Fig. S8 ), the immunofluorescence observation indicated that both endogenous and transgene-derived PLCδ1 protein was expressed in suprabasal epidermis ( Fig. 3d ). These expression patterns were consistent with enriched expression of PLCδ1 and Foxn1 in differentiated keratinocytes [29] , [30] . At the histological level, the introduction of Foxn1::PLCδ1 gene rescued epidermal hyperplasia and immune cell infiltration that were observed in PLCδ1 −/− mice [20] ( Fig. 3e,f ). Importantly, IL-17 expression was remarkably decreased in Tg/KO skin ( Fig. 3g ) compared with PLCδ1 −/− skin. Residual expression of IL-17 mRNA in Tg/KO skin may be caused by a lower level of PLCδ1 protein expression in Tg/KO than in control skin. Tg/KO mice showed no lymphadenopathy of the ILNs ( Fig. 3h , Supplementary Table S2 ), and IL-17-producing cells were not increased in the ILNs in Tg/KO mice ( Fig. 3i,j ). Thus, reintroduction of PLCδ1 into keratinocytes ameliorated local IL-17 upregulation. In addition, IL-17 concentrations in the serum of Tg/KO mice reverted to undetectable levels as in control mice ( Fig. 3k ), strongly suggesting that skin- and skin-draining lymph node-derived IL-17 was required for the elevation of IL-17 levels in serum. We also examined granulocyte populations in the peripheral blood, spleen, and bone marrow. Interestingly, Tg/KO mice did not exhibit granulocytosis ( Fig. 3l ), suggesting a close correlation between granulocytosis and IL-17 levels. These observations indicate that PLCδ1 expression in keratinocytes was sufficient for normal granulocyte counts and IL-17 levels in PLCδ1 −/− mice. 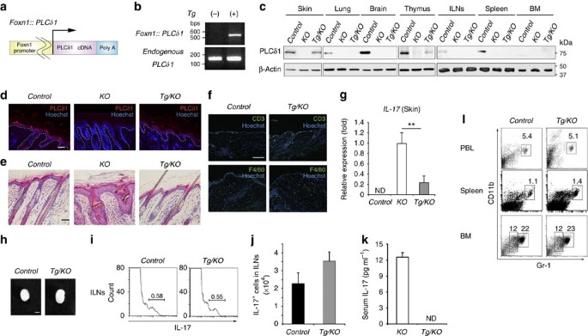Figure 3: Reintroduction of PLCδ1 inPLCδ1−/−keratinocytes restores normal IL-17 levels and granulocyte counts. (a) Structure of theFoxn1::PLCδ1gene. Poly A: the bovine growth hormone polyadenylation sequence. (b) PCR analysis of genomic DNA from the tails ofwild-typeandFoxn1::PLCδ1Tg mice. Products derived fromFoxn1::PLCδ1and endogenousPLCδ1. (c) Immunoblotting of PLCδ1 and β-actin in tissues from control,PLCδ1−/−(KO), andTg/KOmice. (d) Skin stained with antibody against PLCδ1 (red) and Hoechst stain (blue). Dotted lines denote the dermal-epidermal border. Scale bar, 50 μm. (e) Haematoxylin-eosin (HE) stained dorsal skin sections. Scale bar, 50 μm. (f) The skin was stained with antibodies against CD3 (green) or F4/80 (green) and Hoechst (blue). Scale bar, 100 μm. (g)IL-17mRNA expression in the skin of control,PLCδ1−/−(KO), andTg/KOmice determined by real-time RT–PCR. All values are normalized toGAPDH. Results are displayed as arbitrary units (expression in the skin ofKOmice=1). Mean±s.e.m. (n=5). (h) Macroscopic appearance of ILNs in control andTg/KOmice. Scale bar, 1 mm. (i) Representative FACS profiles of intracellular IL-17 in ILNs. Cells were stimulated and intracellular IL-17 was detected (n=4). Three independent experiments were performed. (j) Absolute numbers of IL-17+cells. Mean±s.e.m. (n=4). The combined results from three independent experiments are displayed. (k) IL-17 concentration in serum measured by ELISA. Mean±s.e.m. (n=3). (l) Representative FACS profiles of CD11b+Gr-1+granulocytes in the PBL, spleen, and BM ofTg/KOmice (n=4). (d–l) 8–12-week-old mice were used. (d–j,l) Heterozygotes withFoxn1::PLCδ1were used as controls. Statistical significance was assessed using a Student′st-test. **P<0.01. ND, not detected. Figure 3: Reintroduction of PLCδ1 in PLCδ1 −/− keratinocytes restores normal IL-17 levels and granulocyte counts. ( a ) Structure of the Foxn1::PLCδ1 gene. Poly A: the bovine growth hormone polyadenylation sequence. ( b ) PCR analysis of genomic DNA from the tails of wild-type and Foxn1::PLCδ1 Tg mice. Products derived from Foxn1::PLCδ1 and endogenous PLCδ1 . ( c ) Immunoblotting of PLCδ1 and β-actin in tissues from control, PLCδ1 −/− ( KO ), and Tg/KO mice. ( d ) Skin stained with antibody against PLCδ1 (red) and Hoechst stain (blue). Dotted lines denote the dermal-epidermal border. Scale bar, 50 μm. ( e ) Haematoxylin-eosin (HE) stained dorsal skin sections. Scale bar, 50 μm. ( f ) The skin was stained with antibodies against CD3 (green) or F4/80 (green) and Hoechst (blue). Scale bar, 100 μm. ( g ) IL-17 mRNA expression in the skin of control, PLCδ1 −/− ( KO ), and Tg/KO mice determined by real-time RT–PCR. All values are normalized to GAPDH . Results are displayed as arbitrary units (expression in the skin of KO mice=1). Mean±s.e.m. ( n =5). ( h ) Macroscopic appearance of ILNs in control and Tg/KO mice. Scale bar, 1 mm. ( i ) Representative FACS profiles of intracellular IL-17 in ILNs. Cells were stimulated and intracellular IL-17 was detected ( n =4). Three independent experiments were performed. ( j ) Absolute numbers of IL-17 + cells. Mean±s.e.m. ( n =4). The combined results from three independent experiments are displayed. ( k ) IL-17 concentration in serum measured by ELISA. Mean±s.e.m. ( n =3). ( l ) Representative FACS profiles of CD11b + Gr-1 + granulocytes in the PBL, spleen, and BM of Tg/KO mice ( n =4). ( d – l ) 8–12-week-old mice were used. ( d – j , l ) Heterozygotes with Foxn1::PLCδ1 were used as controls. Statistical significance was assessed using a Student′s t -test. ** P <0.01. ND, not detected. Full size image Epidermal PLCδ1 regulates local and systemic IL-17 levels We examined whether loss of PLCδ1 in keratinocytes caused IL-17 upregulation and granulocytosis by generating keratinocyte-specific conditional PLCδ1 -knockout ( cKO ) mice with K14 promoter-driven Cre transgenic mice ( Fig. 4a,b ). We confirmed that PLCδ1 was deleted in the epidermis of the cKO mice and that its expression was not altered in other organs such as the lungs, brain, ILNs, spleen, and bone marrow ( Fig. 4c ). As the K14 promoter is active in the thymus, we examined the expression of PLCδ1 in the thymus, finding that PLCδ1 was downregulated in the thymus of cKO mice ( Fig. 4c ). However, we did not observe any obvious abnormalities in cKO thymus. IL-17 was upregulated in the skin of cKO mice ( Fig. 4d ), whereas interferon γ and IL-4 expression levels remained unchanged ( Supplementary Fig. S7b ). Interestingly, IL-17 mRNA was upregulated more in the epidermis than in whole skin of cKO mice ( Fig. 4e ). CD3-positive T cells were major IL-17 producers in the cKO epidermis ( Fig. 4f ). The number of CD3-positive T cells was 1.7-fold higher in cKO than in control epidermis, suggesting that upregulation of IL-17 mRNA in cKO epidermis is due, at least in part, to an increase in T cells. Further analysis revealed that IL-17 was expressed by Vγ3-positive γδ T cells in cKO epidermis ( Supplementary Fig. S9a ). We also found that the level of IL-17 mRNA was not significantly altered by depletion of Langerhans cells ( Supplementary Fig. S9b ). cKO mice also showed increased ILN size ( Fig. 4g ; Supplementary Table S3 ) and cell numbers (mean±s.e.m. cell numbers, 3.7±0.9×10 6 in controls versus 14±2.4×10 6 in cKO mice, both n =6). The number of IL-17-producing cells in the ILNs of cKO mice was more than six times that in the control mice ( Fig. 4h ). The main IL-17-producing cells in cKO ILNs were γδ T cells ( Fig. 4i ). IL-17 upregulation in ILNs of cKO mice was also confirmed by real-time RT–PCR ( Fig. 4j ). Production of the granulopoietic cytokine G-CSF is induced by IL-17 in many cell types, and we, therefore, examined whether conditioned medium (CM) derived from cKO skin-draining lymph nodes induced G-CSF expression. CM from cKO skin-draining lymph nodes induced higher G-CSF expression in fibroblasts compared with CM from control skin-draining lymph nodes ( Fig. 4k ). Importantly, CM from cKO skin-draining lymph nodes pretreated with anti-IL-17 neutralizing antibody did not cause G-CSF upregulation ( Fig. 4k ), strongly suggesting that cells in the cKO skin-draining lymph nodes secrete IL-17, leading to G-CSF production. If IL-17 derived from skin and skin-draining lymph nodes causes serum IL-17 elevation, then serum IL-17 concentrations should also be increased in cKO mice. Indeed, serum IL-17 levels were high in cKO mice ( Fig. 4l ), strongly suggesting that local IL-17 upregulation is linked to elevation of serum IL-17 levels. In addition, serum G-CSF concentrations were significantly increased in cKO mice compared with control mice ( Fig. 4m ). We further investigated the granulocyte population in cKO mice and found that cKO mice showed granulocytosis ( Fig. 4n ), consistent with local and serum IL-17 upregulation. Reduced numbers of bone marrow B lymphocytes and erythrocytes were also observed in cKO mice ( Supplementary Fig. S10 ). Taken together, these results indicate that PLCδ1 in keratinocytes is required for the maintenance of normal IL-17 levels and granulocyte counts. 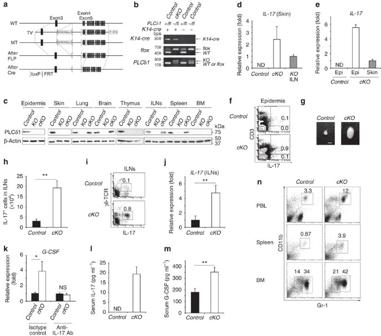Figure 4: Epidermal loss of PLCδ1 results in IL-17 upregulation and granulocytosis. (a) Genomic structure of thePLCδ1gene (WT). Exons are indicated by filled boxes. The structures of the targeting vector (TV) for disrupting the mousePLCδ1, targeted allele (MT), allele after FLP recombination (After FLP), and allele after Cre recombination (After Cre) are displayed. (b) PCR genotyping of control andcKOmice. (c) Immunoblotting of PLCδ1 and β-actin in tissues from control,PLCδ1−/−(KO), andcKOmice. (d)IL-17mRNA expression in skin.KOILN was used as positive control forIL-17expression. Results are displayed as arbitrary units (expression inKOILN=1). Mean±s.e.m. (n=3). (e)IL-17mRNA expression in epidermis (epi) and whole skin (skin). Results are displayed as arbitrary units (expression incKOwhole skin=1). Mean±s.e.m. (n=3). (f) Representative FACS profiles of IL-17 and CD3 of epidermis (n=3). Three independent experiments were performed. (g) Macroscopic appearance of ILNs. Scale bar=2 mm. (h) Absolute numbers of IL-17+cells in ILNs. Mean±s.e.m. (n=6). (i) Representative FACS profiles of γδ-TCR and intracellular IL-17 in ILNs (n=6). Cells were stimulated. Five independent experiments were performed. (j)IL-17mRNA expression in the ILNs. Results are listed as arbitrary units (expression in control mice=1). Mean±s.e.m. (n=3). (k)G-CSFexpression in Swiss 3T3 cells treated with skin-draining lymph-node CM in the presence of anti-IL-17 neutralizing antibody or isotype control. Results are displayed as arbitrary units (expression in cells treated with control skin-draining lymph-node CM and isotype control=1). Mean±s.e.m. (n=4). (l) IL-17 concentration in serum. Mean±s.e.m. (n=10). (m) G-CSF concentration in the serum. Mean±s.e.m. (n=6). (n) Representative FACS profiles of CD11b+Gr-1+granulocytes (n=8). (d,e,j,k) All values are normalized toGAPDH. (d–n) 8–12-week-old mice were used. Statistical significance was assessed using a Student′st-test. *P<0.05; **P<0.01. ND, not detected. Figure 4: Epidermal loss of PLCδ1 results in IL-17 upregulation and granulocytosis. ( a ) Genomic structure of the PLCδ1 gene (WT). Exons are indicated by filled boxes. The structures of the targeting vector (TV) for disrupting the mouse PLC δ 1 , targeted allele (MT), allele after FLP recombination (After FLP), and allele after Cre recombination (After Cre) are displayed. ( b ) PCR genotyping of control and cKO mice. ( c ) Immunoblotting of PLCδ1 and β-actin in tissues from control, PLCδ1 −/− ( KO ), and cKO mice. ( d ) IL-17 mRNA expression in skin. KO ILN was used as positive control for IL-17 expression. Results are displayed as arbitrary units (expression in KO ILN=1). Mean±s.e.m. ( n =3). ( e ) IL-17 mRNA expression in epidermis (epi) and whole skin (skin). Results are displayed as arbitrary units (expression in cKO whole skin=1). Mean±s.e.m. ( n =3). ( f ) Representative FACS profiles of IL-17 and CD3 of epidermis ( n =3). Three independent experiments were performed. ( g ) Macroscopic appearance of ILNs. Scale bar=2 mm. ( h ) Absolute numbers of IL-17 + cells in ILNs. Mean±s.e.m. ( n =6). ( i ) Representative FACS profiles of γδ-TCR and intracellular IL-17 in ILNs ( n =6). Cells were stimulated. Five independent experiments were performed. ( j ) IL-17 mRNA expression in the ILNs. Results are listed as arbitrary units (expression in control mice=1). Mean±s.e.m. ( n =3). ( k ) G-CSF expression in Swiss 3T3 cells treated with skin-draining lymph-node CM in the presence of anti-IL-17 neutralizing antibody or isotype control. Results are displayed as arbitrary units (expression in cells treated with control skin-draining lymph-node CM and isotype control=1). Mean±s.e.m. ( n =4). ( l ) IL-17 concentration in serum. Mean±s.e.m. ( n =10). ( m ) G-CSF concentration in the serum. Mean±s.e.m. ( n =6). ( n ) Representative FACS profiles of CD11b + Gr-1 + granulocytes ( n =8). ( d , e , j , k ) All values are normalized to GAPDH . ( d – n ) 8–12-week-old mice were used. Statistical significance was assessed using a Student′s t -test. * P <0.05; ** P <0.01. ND, not detected. Full size image Epidermal PLCδ1 regulates IL-23 expression in the skin We investigated the mechanisms of IL-17 upregulation in the epidermis by analysing the expression of the IL-17-inducing cytokine, IL-23. IL-23 and IL-12 are functionally related as heterodimeric cytokines that share the IL-12/23p40 subunit [31] . The mRNAs for the subunits of the IL-23 heterodimer ( IL-12/23p40 and IL-23p19 ) were upregulated in cKO skin ( Fig. 5a ), while IL-12p35 , which encodes the IL-12-specific subunit, was not upregulated ( Fig. 5a ). In contrast, a dramatic decrease in IL-23 expression was detected after reintroduction of PLCδ1 into keratinocytes ( Supplementary Fig. S11 ). As Tg/KO skin showed no drastic increase in IL-17 ( Fig. 3g ) whereas cKO skin showed remarkable IL-17 upregulation ( Fig. 4d ), the expression level of IL-23 was closely correlated with that of IL-17 in skin. Similar to IL-17, IL-23p19 mRNA and protein were upregulated in cKO epidermis ( Fig. 5b,c ). Immunofluorescence experiments showed faint IL-23p19 immunoreactivity in control epidermis, whereas keratinocytes in the basal layer of cKO epidermis showed strong IL-23p19 immunoreactivity ( Fig. 5d ). IL-23p19 expression was also assessed in primary keratinocyte cultures. cKO keratinocytes did not show increased expression of IL-23p19 , regardless of their differentiation status ( Fig. 5e ). Thus, loss of PLCδ1 from keratinocytes did not upregulate IL-23 in this in vitro system, suggesting that interactions between PLCδ1-deficient keratinocytes and other epidermal cells may be required for IL-23 production. We then examined whether the epidermal increase in IL-23 was linked to IL-17 upregulation in the cKO epidermis. IL-23 was neutralized using its specific p19 subunit antibody, and IL-17 expression was then examined in control and cKO epidermal sheets. IL-17 mRNA levels in the cKO epidermal sheet were clearly decreased in the presence of anti-IL-23p19 neutralizing antibody, compared with levels in the presence of isotype control ( Fig. 5f ), indicating that IL-23 has a critical role in IL-17 upregulation in cKO epidermis. We then investigated the mechanisms responsible for IL-23 upregulation by assessing activation of PLC and its downstream effector, PKC. We found that overall PLC activity was drastically decreased in cKO compared with control epidermis ( Fig. 5g ), indicating that, even in the presence of other PLC isoforms, loss of PLCδ1 impaired PLC activity in the epidermis. Consistent with the decrease in PLC activity, we found that the phosphorylation of PKC substrates was markedly decreased in cKO epidermis ( Fig. 5h ), indicating that loss of PLCδ1 from keratinocytes impaired the activation of the PLC downstream effector. We next determined whether the PLC downstream signal affected IL-23 expression. PLC activation results in the generation of IP 3 and DAG, leading to elevated concentrations of intracellular calcium ions and activation of PKC. We, therefore, treated epidermal sheets with the calcium ionophore, ionomycin and phorbol 12-myristate 13-acetate (PMA), a synthetic analogue of DAG and a PKC activator, to mimic PLC activation. IL-23p19 expression was upregulated in cKO epidermal sheets in the absence of ionomycin and PMA. Importantly, IL-23p19 upregulation was ameliorated in cKO epidermal sheets in the presence of ionomycin and PMA ( Fig. 5i ). Expression of the IL-12-specific subunit, IL-12p35 , was unchanged in the epidermis, regardless of the presence or absence of ionomycin and PMA ( Fig. 5i ). These results strongly suggest that IL-23 upregulation in the cKO epidermis was caused by impaired PLC downstream signalling. 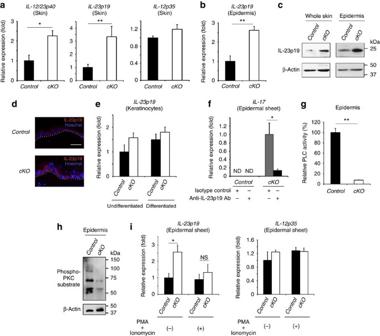Figure 5: IL-23 was upregulated incKOskin. (a)IL-12/23p40,IL-23p19, andIL-12p35mRNA expression in the skin determined by real-time RT–PCR. All values are normalized toGAPDH. Results are displayed as arbitrary units (expression in control skin=1). Mean±s.e.m. (n=5). (b)IL-23p19mRNA expression in epidermis determined by real-time RT–PCR. All values are normalized toGAPDH. Results are displayed as arbitrary units (expression in control=1). Mean±s.e.m. (n=6). (c) Immunoblotting of IL-23p19 and β-actin in whole skin and epidermis from control andcKOmice. (d) Skin stained with the antibody against IL-23p19 (red) and Hoechst (blue). Dotted lines denote dermal-epidermal border. Scale bar, 30 μm. (e)IL-23p19mRNA expression in primary keratinocyte cultures determined by real-time RT–PCR. All values are normalized toGAPDH. Results are displayed as arbitrary units (expression in undifferentiated control keratinocytes=1). Mean±s.e.m. (n=3). (f) Epidermal sheets were treated with anti-IL-23p19 neutralizing antibody or normal goat IgG, andIL-17mRNA expression was determined. All values are normalized toGAPDH. Results are displayed as arbitrary units (expression incKOepidermal sheet treated with isotype control=1). Mean±s.e.m. (n=4). (g) Relative PLC activity in epidermal lysates (PLC activity in control epidermis=100%). Mean±s.e.m. (n=4). (h) Immunoblotting for phospho-PKC substrate in epidermis. β-actin was included as a loading control. (i) Epidermal sheets were treated with PMA and ionomycin, and mRNA expression ofIL-23p19andIL-12p35was determined. All values are normalized toGAPDH. Results are displayed as arbitrary units (expression in control epidermal sheet without PMA/ionomycin treatment=1). Mean±s.e.m. (n=4). Mice used in all experiments were 8–12 weeks old. Statistical significance was assessed using a Student′st-test. *P<0.05; **P<0.01. ND, not detected; NS, not significant. Figure 5: IL-23 was upregulated in cKO skin. ( a ) IL-12/23p40 , IL-23p19 , and IL-12p35 mRNA expression in the skin determined by real-time RT–PCR. All values are normalized to GAPDH . Results are displayed as arbitrary units (expression in control skin=1). Mean±s.e.m. ( n =5). ( b ) IL-23p19 mRNA expression in epidermis determined by real-time RT–PCR. All values are normalized to GAPDH . Results are displayed as arbitrary units (expression in control=1). Mean±s.e.m. ( n =6). ( c ) Immunoblotting of IL-23p19 and β-actin in whole skin and epidermis from control and cKO mice. ( d ) Skin stained with the antibody against IL-23p19 (red) and Hoechst (blue). Dotted lines denote dermal-epidermal border. Scale bar, 30 μm. ( e ) IL-23p19 mRNA expression in primary keratinocyte cultures determined by real-time RT–PCR. All values are normalized to GAPDH . Results are displayed as arbitrary units (expression in undifferentiated control keratinocytes=1). Mean±s.e.m. ( n =3). ( f ) Epidermal sheets were treated with anti-IL-23p19 neutralizing antibody or normal goat IgG, and IL-17 mRNA expression was determined. All values are normalized to GAPDH . Results are displayed as arbitrary units (expression in cKO epidermal sheet treated with isotype control=1). Mean±s.e.m. ( n =4). ( g ) Relative PLC activity in epidermal lysates (PLC activity in control epidermis=100%). Mean±s.e.m. ( n =4). ( h ) Immunoblotting for phospho-PKC substrate in epidermis. β-actin was included as a loading control. ( i ) Epidermal sheets were treated with PMA and ionomycin, and mRNA expression of IL-23p19 and IL-12p35 was determined. All values are normalized to GAPDH . Results are displayed as arbitrary units (expression in control epidermal sheet without PMA/ionomycin treatment=1). Mean±s.e.m. ( n =4). Mice used in all experiments were 8–12 weeks old. Statistical significance was assessed using a Student′s t -test. * P <0.05; ** P <0.01. ND, not detected; NS, not significant. Full size image cKO skin shares features of human inflammatory skin diseases Because patients with human inflammatory skin diseases, such as psoriasis, show upregulation of IL-23 and IL-17 in the skin [8] , [32] , [33] , PLCδ1 could be involved in pathogenesis of these diseases. We therefore, examined PLCδ1 expression in the topical imiquimod (IMQ)-induced psoriasiform lesion, which is a mouse model of human psoriasis [34] . Interestingly, PLCδ1 protein was decreased in IMQ-treated skin compared with non-treated skin ( Fig. 6a ). PLCδ1 downregulation was also observed in the epidermis of IMQ-treated mice ( Fig. 6a ). These observations strongly suggest that epidermal PLCδ1 is implicated in a mouse model of human psoriasis. We next determined whether cKO skin shares features of human inflammatory skin diseases. Histological analysis revealed that cKO skin showed acanthosis ( Fig. 6b ) and infiltration of immune cells ( Fig. 6c ), as seen in human inflammatory skin diseases, such as psoriasis. In addition, cKO epidermis displayed abnormal patterns of differentiation marker expression, including the interfollicular expression of K6 ( Supplementary Fig. S12 ), which is observed in human inflammatory skin diseases. Real-time RT–PCR showed that inflammatory genes upregulated in human inflammatory skin diseases are also upregulated in cKO skin ( Fig. 6d ) [35] , [36] , [37] , [38] , [39] , [40] . Activation of the signal transducer and activator of transcription 3 (STAT3) is also a feature of psoriasis [41] , and western blotting revealed that both total and phosphorylated STAT3 proteins were increased in cKO skin ( Fig. 6e ). Consistent with these results, immunohistochemistry detected phosphorylated STAT3 in the nuclei of the cKO epidermis ( Fig. 6f ). Because the dermis is highly vascularized in some skin diseases [42] , [43] , [44] , [45] , we analysed the expression levels of the potent angiogenic factor, vascular endothelial growth factor (VEGF ). VEGF upregulation was observed in cKO skin ( Fig. 6g ). In addition, immunofluorescence revealed that cKO skin was highly vascularized ( Fig. 6h ), in a manner similar to that in human inflammatory skin diseases. Most phenotypes in cKO skin were also observed in a mouse model of human psoriasis ( Supplementary Fig. S13 ). Interestingly, PLCδ1 protein was downregulated in epidermis of human psoriatic skin ( Fig. 6i ). These observations strongly suggest that epidermal PLCδ1 is involved in human psoriasis. 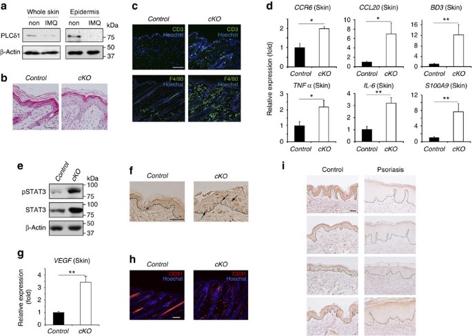Figure 6:cKOskin exhibits features of human inflammatory skin disease. (a) Immunoblotting of PLCδ1 and β-actin in whole skin or epidermis from non-treated (non) or IMQ-treated (IMQ) mice. (b) HE stained dorsal skin sections. Scale bar, 50 μm. The control skin has a normal epidermis, whereas the cKO skin has a thickened epidermis. (c) The skin was stained with antibodies against CD3 (green) or F4/80 (green) and Hoechst (blue). Scale bar,100 μm. (d)CCR6,CCL20,β-defensin3(BD3),TNF α,IL-6, andS100A9mRNA expression in skin determined by real-time RT–PCR. All values are normalized toGAPDH. Results are displayed as arbitrary units (expression in skin of control mice=1). Mean±s.e.m. (n=5). (e) Immunoblotting for total and phosphorylated STAT3 (pSTAT3) in skin. β-actin was included as a loading control. (f) Skin stained with antibody against phosphorylated STAT3. Dotted lines denote dermal–epidermal border. Scale bar, 20 μm. Nuclear staining of phosphorylated STAT3 is indicated by arrows. (g)VEGFmRNA expression in skin determined by real-time RT–PCR. All values are normalized toGAPDH. Results are displayed as arbitrary units (expression in skin of control mice=1). Mean±s.e.m. (n=5). (h) Skin stained with the antibody against CD31 (red) and Hoechst (blue). Hair shafts show nonspecific auto-fluorescence (red). Scale bar, 100 μm. (i) Skin from four non-psoriatic volunteers and four patients with psoriasis were stained with antibody against human PLCδ1 (brown). Dotted lines denote dermal–epidermal border. Scale bar, 100 μm. Body sites of each skin samples were as follows: control; arm, waist, back, and back (indicated from the top panel to the bottom panel). Psoriasis; arm, abdominal, leg, and leg (indicated from the top panel to the bottom panel). (a,c–h) 8–12-week-old mice were used. (b–h) Untreated IMQs were used. The data presented in (b,c,e,f,h) are representative of analyses of three mice per genotype. The data presented in (a) is representative of analyses of two mice per genotype. Statistical significance was assessed using a Student′st-test. *P<0.05; **P<0.01. Figure 6: cKO skin exhibits features of human inflammatory skin disease. ( a ) Immunoblotting of PLCδ1 and β-actin in whole skin or epidermis from non-treated (non) or IMQ-treated (IMQ) mice. ( b ) HE stained dorsal skin sections. Scale bar, 50 μm. The control skin has a normal epidermis, whereas the cKO skin has a thickened epidermis. ( c ) The skin was stained with antibodies against CD3 (green) or F4/80 (green) and Hoechst (blue). Scale bar,100 μm. ( d ) CCR6 , CCL20 , β-defensin3 ( BD3 ), TNF α , IL-6 , and S100A9 mRNA expression in skin determined by real-time RT–PCR. All values are normalized to GAPDH . Results are displayed as arbitrary units (expression in skin of control mice=1). Mean±s.e.m. ( n =5). ( e ) Immunoblotting for total and phosphorylated STAT3 (pSTAT3) in skin. β-actin was included as a loading control. ( f ) Skin stained with antibody against phosphorylated STAT3. Dotted lines denote dermal–epidermal border. Scale bar, 20 μm. Nuclear staining of phosphorylated STAT3 is indicated by arrows. ( g ) VEGF mRNA expression in skin determined by real-time RT–PCR. All values are normalized to GAPDH . Results are displayed as arbitrary units (expression in skin of control mice=1). Mean±s.e.m. ( n =5). ( h ) Skin stained with the antibody against CD31 (red) and Hoechst (blue). Hair shafts show nonspecific auto-fluorescence (red). Scale bar, 100 μm. ( i ) Skin from four non-psoriatic volunteers and four patients with psoriasis were stained with antibody against human PLCδ1 (brown). Dotted lines denote dermal–epidermal border. Scale bar, 100 μm. Body sites of each skin samples were as follows: control; arm, waist, back, and back (indicated from the top panel to the bottom panel). Psoriasis; arm, abdominal, leg, and leg (indicated from the top panel to the bottom panel). ( a , c – h ) 8–12-week-old mice were used. ( b – h ) Untreated IMQs were used. The data presented in ( b , c , e , f , h ) are representative of analyses of three mice per genotype. The data presented in ( a ) is representative of analyses of two mice per genotype. Statistical significance was assessed using a Student′s t -test. * P <0.05; ** P <0.01. Full size image PLCδ1 in keratinocytes influences contact hypersensitivity Dinitrofluorobenzene (DNFB)-induced contact hypersensitivity (CHS) of the skin in mice is commonly used as a model for studying the pathogenesis of allergic contact dermatitis (ACD), in which IL-17 has a critical role [4] , [46] . We, therefore, assessed CHS responses in cKO mice. Mice were sensitized and challenged with DNFB, and the CHS response was assessed by measuring ear swelling. On challenge with DNFB, DNFB-sensitized control mice exhibited a CHS response with mild ear swelling, whereas cKO mice showed more prominent ear swelling with exaggerated edema and severe inflammatory cell infiltration ( Fig. 7a,b ). Interestingly, IL-17 neutralization resulted in abrogation of the exaggerated ear swelling in cKO mice almost to basal level at any time after challenge ( Fig. 7c ). These results indicate that the exacerbated CHS in cKO mice was IL-17-dependent. 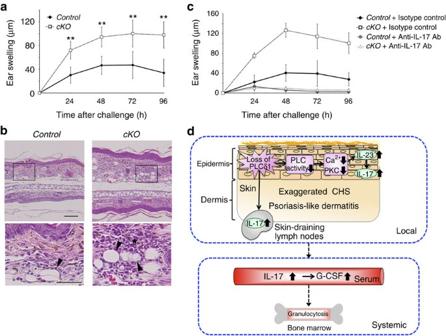Figure 7: Loss of PLCδ1 in keratinocytes exaggerates CHS responses. (a) Time course of ear swelling after DNFB challenge. Ear swelling was measured at the indicated times. Mean±s.d. (n=4). (b) HE stains of ear after DNFB challenge. The ears of sensitized mice were painted with DNFB, collected 96 h later and stained with HE. Lower panels are magnified views of the boxed regions in the upper panels. Scale bar in upper panel, 100 μm. Scale bar in lower panel,50 μm. (c) Sensitized mice were treated with anti-IL-17 neutralizing antibody or normal rat IgG before challenge, and ear swelling was measured at the indicated times. Mean±s.d. (n=3). Mice used in all experiments were 8–12 weeks old. The data presented in (b) are representative of three mice per genotype. Statistical significance was assessed using a Student′st-test. **P<0.01. (d) Proposed model of local and systemic phenotypes induced by epidermal loss of PLCδ1. Epidermal loss of PLCδ1 impairs overall PLC activity and activation of PLC downstream signals, which causes increased production of IL-23 in the epidermis and whole skin. IL-23 induces IL-17 production in the epidermis. IL-17 was also overproduced in the skin-draining lymph nodes. This aberrant activation of the local IL-23/IL-17 axis resulted in a phenotype similar to that in human psoriasis and exaggerated CHS responses. Regarding systemic phenotypes, serum IL-17 levels were increased presumably as a result of skin and/or skin-draining lymph node-derived IL-17 (dotted arrow). Elevated serum IL-17 concentrations likely cause subsequent granulocytosis through G-CSF production (dotted arrow). Figure 7: Loss of PLCδ1 in keratinocytes exaggerates CHS responses. ( a ) Time course of ear swelling after DNFB challenge. Ear swelling was measured at the indicated times. Mean±s.d. ( n =4). ( b ) HE stains of ear after DNFB challenge. The ears of sensitized mice were painted with DNFB, collected 96 h later and stained with HE. Lower panels are magnified views of the boxed regions in the upper panels. Scale bar in upper panel, 100 μm. Scale bar in lower panel,50 μm. ( c ) Sensitized mice were treated with anti-IL-17 neutralizing antibody or normal rat IgG before challenge, and ear swelling was measured at the indicated times. Mean±s.d. ( n =3). Mice used in all experiments were 8–12 weeks old. The data presented in ( b ) are representative of three mice per genotype. Statistical significance was assessed using a Student′s t -test. ** P <0.01. ( d ) Proposed model of local and systemic phenotypes induced by epidermal loss of PLCδ1. Epidermal loss of PLCδ1 impairs overall PLC activity and activation of PLC downstream signals, which causes increased production of IL-23 in the epidermis and whole skin. IL-23 induces IL-17 production in the epidermis. IL-17 was also overproduced in the skin-draining lymph nodes. This aberrant activation of the local IL-23/IL-17 axis resulted in a phenotype similar to that in human psoriasis and exaggerated CHS responses. Regarding systemic phenotypes, serum IL-17 levels were increased presumably as a result of skin and/or skin-draining lymph node-derived IL-17 (dotted arrow). Elevated serum IL-17 concentrations likely cause subsequent granulocytosis through G-CSF production (dotted arrow). Full size image In all of our mouse models, the level of expression of PLCδ1 in keratinocytes was inversely correlated with the levels of expression of IL-23 and IL-17 in skin and skin-draining LNs. Thus, loss of PLCδ1 in keratinocytes results in local activation of the IL-23/IL-17 axis ( Fig. 7d ). Keratinocytes from lesional psoriatic skin express IL-23 (ref. 32 ). In addition, human keratinocytes stimulated with nickel, a common hapten inducing CHS, produce IL-23 (ref. 47 ). These results are consistent with our observation that IL-23p19 was upregulated in keratinocytes of cKO epidermis ( Fig. 5d ). Because IL-23p19 was upregulated mainly in basal layer of cKO interfollicular epidermis ( Fig. 5d ), essential and sufficient roles of suprabasal PLCδ1 in maintenance of normal IL-23p19 levels ( Fig. 3d ; Supplementary Fig. S11 ) is somewhat surprising. Interactions between suprabasal and basal keratinocytes might be important in regulation of IL-23p19 expression. We also found that γδ T cells in cKO epidermis expressed IL-17 ( Supplementary Fig. S9 ). Interestingly, γδ T cells were recently reported to be major IL-17 producers in skin of IL-23-mediated psoriasiform dermatitis [48] , [49] . Aberrant activation of the IL-23/IL-17 axis in the skin is known to be involved in the development of inflammatory human skin diseases, especially psoriasis [8] . Indeed, IL-23 injection into normal skin was sufficient for the development of psoriatic phenotypes in mice [50] , [51] , and a monoclonal antibody against IL-12/23p40 subunit, ustekinumab is efficacious for the treatment of patients with moderate-to-severe psoriasis [52] . Although cKO skin shared some molecular features of psoriasis, it did not demonstrate all the histological characteristics of psoriatic skin. This may be because the expression of another key cytokine for the development of psoriasis, IL-22, was not upregulated in cKO skin (data not shown). Nonetheless, as PLCδ1 expression was decreased in the epidermis of patients with psoriasis ( Fig. 6i ) and in mouse IMQ-induced psoriasiform lesion ( Fig. 6a ), PLCδ1 may be involved in the pathogenesis of psoriasis. cKO mice also demonstrated increased sensitivity to hapten-induced CHS, a mouse model of human ACD. The fact that the exaggerated CHS response in cKO mice was inhibited by IL-17 neutralization demonstrated the involvement of PLCδ1 in IL-17-mediated ACD. Keratinocyte-specific ablation of PLCδ1 also caused systemic elevation of IL-17 and granulocytosis. Because activation of the local IL-23/IL-17 axis and systemic granulocytosis were both observed in cKO , but not in Tg/KO mice, the absence of epidermal PLCδ1, local IL-23/IL-17 axis activation, and systemic granulocytosis were strongly correlated with each other. This strict correlation strongly suggests that activation of the local IL-23/IL-17 axis and elevation of serum IL-17 and G-CSF concentrations are likely to be responsible for granulocytosis. On the basis of previous findings [53] , the serum concentrations of IL-17 and G-CSF in PLCδ1 −/− and cKO mice were sufficient to produce a systemic increase in granulocytes. The loss of JunB in keratinocytes was recently reported to cause a myeloproliferative disease characterized by increased granulocytes through elevated G-CSF production by keratinocytes [54] . As expression levels of JunB and G-CSF were unaltered in epidermis of cKO mice (data not shown), PLCδ1 seems to cause granulocytosis by a different mechanism to that observed in keratinocyte-specific JunB -knockout mice. The results of this study demonstrate that disruption of the PLCδ1 gene in keratinocytes disturbs not only local skin immune responses, but also the systemic homeostasis of haematopoietic cells, especially granulocytes. The proposed mechanism underlying the phenotypes seen in cKO mice is depicted in Fig. 7d . These findings suggest that targeting body-surface-specific inflammatory pathways may prevent not only inflammatory skin diseases but systemic granulocytosis and related disorders too. Mice PLCδ1 −/− mice and PLCδ1 flox/flox mice (Acc. No. CDB0552K: http://www.cdb.riken.jp/arg/mutant%20mice%20list.html) were produced as described [55] ( http://www.cdb.riken.jp/arg/Methods.html ). In brief, a floxed allele of PLCδ1 was generated by inserting loxP sites upstream of exon 4 and downstream of exon 5. The resulting mutant mice carrying the floxed allele of PLCδ1 were crossed with B6-Tg (CAG-FLPe)36 mice (RIKEN BRC, RBRCO 1834) to remove the neomycin-resistant cassette, and then with K14-Cre transgenic mice [56] (#004782, Jackson Laboratory, Bar Harbor, ME, USA) to remove the floxed exons. Foxn1::PLCδ1 transgenic mice (Acc. No. CDB0437T: http://www.cdb.riken.jp/arg/TG%20mutant%20mice%20list.html) were developed as per a standard protocol. In brief, murine PLCδ1 was subcloned into a plasmid that contained a 27,970-bp Foxn1 promoter fragment (gift from Dr T. Boehm) [57] . The construct was linearized and injected into C57BL/6N or BDF1 pronuclei according to standard protocols. Tg/KO mice were generated with two independent transgenic mouse lines. Adult mice or pups were routinely genotyped by PCR. The primer sequences used are listed in Supplementary Table S4 . Age- and sex-matched littermates were used to minimize any effects of genetic background. All animal studies were approved by the animal experiments review board of Tokyo University of Pharmacy and Life Sciences. FACS analysis of cells from peripheral blood and tissues Fluorophor-conjugated monoclonal antibodies were used in various combinations to stain peripheral blood mononuclear cells, splenocytes, and bone marrow. Red blood cells were depleted with 1×RBC Lysis Buffer (eBioscience, San Diego, CA, USA). For staining, 2–5×10 6 cells were used. Fc receptor was blocked by CD16/32 antibody. After staining ( Supplementary Table S5 ), the cells were fixed with 1% paraformaldehyde. Stained and fixed cells were assayed using a FACSCanto flow cytometer (BD Biosciences) and further analysed with FlowJo software (Tree Star, Ashland, OR, USA). BrdU incorporation assay Analysis of in vivo BrdU incorporation into immature granulocytes was performed using the BrdU Flow Kit (BD Pharmingen) after intraperitoneal injection of 1.5 mg of BrdU. Mice were killed 1 h later and the bone marrow cells were collected. Cell surface markers were identified using Gr-1 and CD11b antibodies. Colony-forming unit assays Colony-forming cell assays were performed using bone marrow cells and MethoCult M3434 (Stem Cell Technologies, Vancouver, British Columbia, Canada). Colonies were counted after 12 days' incubation in a humidified atmosphere with 5% CO 2 and characterized according to their unique morphologies. Bone marrow transplantation Recipient mice were irradiated with 9 Gy whole-body irradiation. Donors were PLCδ1 +/− or PLCδ1 −/− (CD45.2 + ) mice, while recipients were of B6.SJL (CD45.1 + ) background. A total of 4×10 6 donor bone marrow cells were intravenously injected into each recipient. Peripheral blood, spleen, and bone marrow chimerism were analysed by immunostaining for CD45 congenic marker isoforms in leukocytes 1 month after transplantation. Intracellular IL-17 staining Cells from ILNs and MLNs were cultured for 4 h in RPMI-1640 (Invitrogen) containing 10% fetal bovine serum (FBS) in the presence of PMA (50 ng ml −1 ; Sigma) and ionomycin (1 μg ml −1 ; Invitrogen). Brefeldin A (10 μg ml −1 ; Sigma) was added for the last 2 h of incubation. Cells were collected and stained with antibodies ( Supplementary Table S5 ) against cell surface antigens. The cells were then subjected to intracellular cytokine staining using the mouse Foxp3 buffer set (BD Pharmingen), according to the manufacturer's instructions. Enzyme-linked immunosorbent assays (ELISA) Serum G-CSF and IL-17 levels were determined using the Quantikine Mouse G-CSF and IL-17 Immunoassay kits (R&D Systems, Minneapolis, MN, USA), respectively, according to the manufacturer's instructions. Real-time RT–PCR Total RNA was isolated using the RNeasy Mini kit (Qiagen, Hilden, Germany), according to the manufacturer's protocol. Template complementary DNA was synthesized from total RNA using the QuantiTect Reverse Transcription kit (Qiagen) or the ReverTra Ace qPCR RT kit (Toyobo, Osaka, Japan). Real-time PCR was performed using the THUNDERBIRD SYBR qPCR Mix (Toyobo) in a CFX96 thermocycler (Bio-Rad, München, Germany). Primer sequences are listed in Supplementary Table S4 . The relative amounts of mRNA were normalized to glyceraldehyde 3-phosphate dehydrogenase mRNA. Immunofluorescence and immunohistochemistry Immunofluorescence analysis for IL-23p19, CD3, F4/80, CD31, K1, K5, K6, and Loricrin was performed using frozen sections. Briefly, sections were fixed in acetone (for IL-23p19) or 2% paraformaldehyde (for CD3, F4/80, CD31, K1, K5, K6 and Loricrin), and nonspecific binding sites were blocked with TNB (PerkinElmer, Waltham, MA, USA). The sections were then incubated with primary antibodies ( Supplementary Table S5 ). Antibody binding was detected by subsequent incubation of the sections with Alexa Fluor 488 or 568-conjugated secondary antibody. Counter-staining was performed with Hoechst 33258 (Invitrogen). Immunofluorescence analysis of mouse PLCδ1 was performed using paraffin sections with TSA Plus Cyanine 3 System (PerkinElmer). Sections were observed under a BZ-8000 microscope (Keyence, Tokyo, Japan). Immunohistochemistry for phosphorylated STAT3 was carried out on paraffin sections, according to the manufacturer's instructions. Immunohistochemical assays for human PLCδ1 were performed using paraffin sections with a Vectastain Elite rabbit ABC kit (Vector Laboratories, Burlingame, CA, USA). Sections were examined under a BX51 microscope (Olympus, Tokyo, Japan). Measurement of PLC activity Epidermis was homogenized in 40 mM HEPES-KOH, pH 7.0, 120 mM KCl containing 0.1% sodium deoxycholate. The PLC activity of these epidermal lysates was assayed by hydrolysis of PI(4,5)P 2 in a 50-μl reaction mixture containing 20,000 d.p.m. of [3H]PI(4,5)P2 (PerkinElmer Life Sciences), 40 μM PI(4,5)P 2 , and 50 μM phosphatidylethanolamine as phospholipids micelles. The micelles were incubated with epidermal lystaes at 37 °C for 5 min, and the reaction was stopped by adding chloroform/methanol (2:1, v/v). Radioactive IP 3 was extracted with 1 N HCl, and radioactivity in the upper aqueous phase was measured for 1 min in a liquid scintillation counter [58] . Hapten-induced CHS Mice were sensitized with DNFB (Sigma) by painting the shaved dorsal skin with 50 μl of 0.5% (w/v) DNFB dissolved in acetone:olive oil (4:1). Five days later, 10 μl of 0.2% (w/v) DNFB was applied to both sides of the right ear. The same volume of acetone:olive oil (4:1) was applied to the left ear as an unchallenged control. Ear swelling was calculated by subtracting the thickness of the left ear from that of the right ear after measurement with a pair of callipers. To detect the role of IL-17 in the elicitation of CHS, mice were sensitized and treated twice intraperitoneally with anti-IL-17 antibody (R&D Systems) (200 μg per mouse) or normal rat IgG (R&D Systems) (200 μg per mouse) on days 4 and 5, after sensitization. Mice were challenged on day 5 and CHS was measured. Explant culture of epidermal sheet Ear or tail skin was removed from adult mice and incubated for 30 min at 37 °C in 0.25% trypsin (Invitrogen) to separate the epidermis from the dermis. For stimulation with PMA and ionomycin, epidermal sheets were cultured for 6 h in RPMI-1640 containing 10% FBS with or without PMA (100 ng ml −1 ) and ionomycin (2.5 μg ml −1 ). For IL-23 neutralization, epidermal sheets were cultured for 24 h in RPMI-1640 containing 10% FBS with 4 μg of anti-IL-23p19 antibody (R&D Systems) or normal goat IgG (R&D Systems). G-CSF induction Swiss 3T3 cells were maintained in DMEM containing 10% FBS. Cells isolated from skin-draining lymph nodes were cultured for 48 h in RPMI-1640 containing 10% FBS and CM was collected. Swiss 3T3 cells were cultured for 24 h in DMEM containing 10% FBS and skin-draining lymph-node CM. Skin-draining lymph-node CM was preincubated with anti-IL-17 antibody (1 μg ml −1 ) or normal rat IgG for 1 h before adding to Swiss 3T3 cells. Intracellular IL-17 staining of epidermal single-cell preparation Ear skin was removed from adult mice and incubated for 1 h at 37 °C in 0.5% trypsin to separate the epidermis from the dermis. Single-cell suspensions were prepared from the epidermis by incubation for an additional 15 min with 0.5% trypsin. Leukocyte enrichment was performed by overlaying a single-cell suspension on a Percoll density gradient and centrifuging. Epidermal cell suspensions were then stained with antibodies against CD3, and the cells were subjected to intracellular IL-17 staining using the mouse Foxp3 buffer set, according to the manufacturer's instructions. IMQ treatment Balb/c mice were treated on the shaved back skin or inner side of the right ear with a daily topical dose of 62.5 or 12.5 mg of commercially available IMQ cream (5%) (Beselna Cream; Mochida Pharmaceuticals, Tokyo, Japan) for 6 days, respectively. Left ears were untreated and used as control. Back skin or ears were collected 24 h after the last treatment. For the preparation of epidermal samples, ear skin was incubated for 30 min at 37 °C in 0.25% trypsin to separate the epidermis from the dermis. Human subjects Patients with psoriasis and healthy volunteers without psoriasis were enrolled. Informed consent was obtained from all participants. The study protocol was approved by the Ethics Committee of Kyoto University and was conducted according to the Declaration of Helsinki Principles. Skin biopsies were analysed by immunohistochemistry. How to cite this article: Kanemaru, K. et al . Epidermal phospholipase Cδ1 regulates granulocyte counts and systemic interleukin-17 levels in mice. Nat. Commun. 3:963 doi: 10.1038/ncomms1960 (2012).